Tcf3 promotes cell migration and wound repair through regulation of lipocalin 2 Cell migration is an integral part of re-epithelialization during skin wound healing, a complex process involving molecular controls that are still largely unknown. Here we identify a novel role for Tcf3, an essential transcription factor regulating embryonic and adult skin stem cell functions, as a key effector of epidermal wound repair. We show that Tcf3 is upregulated in skin wounds and that Tcf3 overexpression accelerates keratinocyte migration and skin wound healing. We also identify Stat3 as an upstream regulator of Tcf3. We show that the promigration effects of Tcf3 are non-cell autonomous and occur independently of its ability to interact with β-catenin. Finally, we identify lipocalin-2 as the key secreted factor downstream of Tcf3 that promotes cell migration in vitro and wound healing in vivo . Our findings provide new insights into the molecular controls of wound-associated cell migration and identify potential therapeutic targets for the treatment of defective wound repair. Cutaneous wound repair is an essential regenerative process, which is required to maintain the barrier function of the skin after damage. This regenerative process is complex with multiple steps that require dynamic interaction of many cell types [1] . Wound healing proceeds in three partially overlapping phases: inflammation, re-epithelialization and tissue remodelling. In the re-epithelialization step, epidermal cells migrate into the wound site, proliferate and differentiate to reform the epidermal barrier. Defects in cell migration often lead to defective wound repair [2] , [3] , [4] , [5] , [6] , [7] . Despite the importance of the re-epithelialization step in the wound healing process, our understanding of the molecular control of this crucial step is still lacking. Tcf3 (also known as Tcf7l1) belongs to the Lef/Tcf family of transcription factors, all of which contain a highly conserved HMG domain that binds to a conserved recognition sequence, as well as domains that interact with the transcriptional activator β-catenin and Groucho/TLE-family corepressors. Lef/Tcf members can function as repressors when bound to Groucho/TLE corepressors or as activators when bound to β-catenin [8] , [9] . In the absence of Wnt ligand, cytoplasmic β-catenin is phosphorylated by the Apc/Axin complex and targeted for degradation. Binding of Wnt ligands to their surface receptors results in the sequestration of components of the Apc/Axin complex, preventing degradation of β-catenin and allowing its translocation into the nucleus. In most cases, nuclear β-catenin interacts with Lef/Tcf members to activate transcription, converting them from corepressors into coactivators. Tcf3 seems to be distinct from the other Lef/Tcf members. Although Tcf3 can bind to β-catenin, its major function throughout development appears to be Groucho/TLE-dependent corepression of transcription [10] , [11] , [12] , [13] , [14] . Tcf3 is expressed in many types of stem cells including embryonic stem cells [11] , [15] and adult hematopoietic [16] , [17] , neural [16] , [18] and skin stem cells [19] , [20] . Loss of function of Tcf3 leads to gastrulation defects and embryonic lethality [21] . In skin, Tcf3 is expressed in embryonic epidermal cells and adult quiescent stem cells located in the hair follicle bulge region, as well as proliferative migrating stem cell progeny [19] , [20] . Overexpression of Tcf3 in the epidermis blocks terminal differentiation and maintains cells in an undifferentiated state [20] , [22] . The expression pattern of Tcf3 in skin is mirrored by its closely related paralog Tcf4 (also known as Tcf7l2), which appears to possess similar functions and can compensate for the absence of Tcf3 in skin development. Loss of both Tcf3 and Tcf4 in skin results in hair follicle morphogenesis defects, as well as failure of re-epithelialization during wound repair and a loss of long-term proliferation/self-renewal [23] . Because the re-epithelialization process during wound repair depends on cell proliferation as well as migration, it is not clear whether Tcf3 has a role in controlling cell migration in addition to its established role in cell proliferation. Tcf3 has been reported to be upregulated in day 26 post-wounded skin [24] , and overexpression of Snail1, which promotes cell migration, also induces Tcf3 expression [25] . Although these two correlative findings suggest that Tcf3 might play a role in wound repair and cell migration, Tcf3’s exact role in cell migration and wound repair is not well understood. In this study, we aim to investigate the role of Tcf3 in wound repair. We find that Tcf3 promotes epidermal cell migration and accelerates wound healing. We also show that Tcf3’s induction in response to wound stimuli is dependent on Stat3, a transcription factor that has previously been shown to be required for efficient wound repair. Moreover, we demonstrate that the pro-migration effects of Tcf3 are non-cell autonomous and occur independently of its ability to interact with the canonical Wnt effector β-catenin. Finally, we identify lipocalin 2 (Lcn2) as the critical downstream target of Tcf3 that promotes cell migration and wound healing. Together, our data delineate a novel Stat3-Tcf3-Lcn2 axis in wound repair. Tcf3 is induced at the wound edge Since the re-epithelialization process is defective in skin lacking Tcf3 and Tcf4, to explore Tcf3’s role in wound healing, we first examined the expression pattern of Tcf3 following full-thickness skin wounding in young adult mice. Within 3 days after wounding, Tcf3 is detectable at the wound edge in K5 positive cells, with maximal expression levels by day 5 ( Fig. 1a ). As expected, Tcf3 is not detectable at the wound edge in Tcf3 conditional knockout skin. We examined other Lef/Tcf members at the wound edge, and found that Tcf4, which has a similar expression pattern to Tcf3 in skin [23] , is also expressed at the wound edge, while Lef1 and Tcf1 (also known as Tcf7), which have dissimilar expression patterns and functions to Tcf3 in adult skin, are unaffected by wounding ( Supplementary Fig. 1 ). 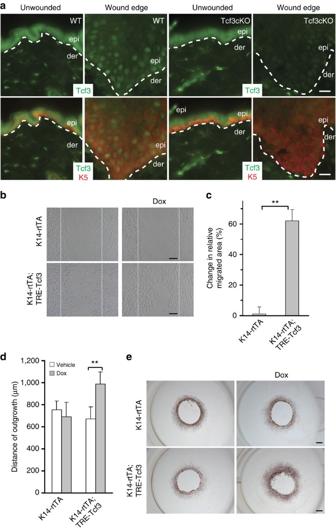Figure 1: Tcf3 is induced at the wound edge and its overexpression promotes cell migration. (a) Images of immunofluorescence analysis of wounded and unwounded skins of WT andTcf3cKO skins. Full-thickness wounds were created on dorsal skins of 10-week-old mice and isolated 5 days post wounding. Skins were analysed by immunofluorescence with antibodies against Tcf3 (green) and keratin 5 (red). Wound-distant skin samples from the same mice were used as unwounded controls. Scale bar, 20 μm. (b) Images of keratinocytes 16 h after the initiation of migration assay. Primary keratinocytes were isolated from tet-inducible Tcf3 (K14rtTA;TRE-Tcf3)or control (K14-rtTA)mice, grown to confluence, treated with Dox or vehicle 24 h prior to being subjected to the migration assay. Cells were treated with mitomycin C for 2 h to arrest proliferation, and a scratch was then made in the confluent monolayer using a pipette tip. The size of the scratch was measured at the beginning of the experiment and the area of cell migration was quantified after 16 h using ImageJ software. Black bar denotes 200 μM. (c) Graph quantifying the area migrated by cells treated with Dox relative to the area migrated by cells treated with vehicle control. For each sample, over 30 non-overlapping fields were measured at each time point; and each experiment was repeated twice. Data are the mean±s.d. **P<0.001 (Student’st-test). (d) Graph quantifying the distance of outgrowth (μm) of epithelial cells from skin explants from control (K14-rtTA)or tet-inducible Tcf3 mice (K14-rtTA;TRE-Tcf3). Dorsal skin punches (4 mm)were cultured for 8 days in the presence or absence of Dox and proliferation was blocked by mitomycin C treatment on day 3. Explants from a minimum of four mice were analysed for each condition. Data are mean±s.d. **P<0.01 (Student’st-test). (e) Representative images of epithelial outgrowth from explants that were immunostained with keratin 17 antibody and counterstained with hematoxylin after 8 days in culture. Scale bar, 1 mm. Figure 1: Tcf3 is induced at the wound edge and its overexpression promotes cell migration. ( a ) Images of immunofluorescence analysis of wounded and unwounded skins of WT and Tcf3 cKO skins. Full-thickness wounds were created on dorsal skins of 10-week-old mice and isolated 5 days post wounding. Skins were analysed by immunofluorescence with antibodies against Tcf3 (green) and keratin 5 (red). Wound-distant skin samples from the same mice were used as unwounded controls. Scale bar, 20 μm. ( b ) Images of keratinocytes 16 h after the initiation of migration assay. Primary keratinocytes were isolated from tet-inducible Tcf3 ( K14rtTA;TRE-Tcf3) or control ( K14-rtTA) mice, grown to confluence, treated with Dox or vehicle 24 h prior to being subjected to the migration assay. Cells were treated with mitomycin C for 2 h to arrest proliferation, and a scratch was then made in the confluent monolayer using a pipette tip. The size of the scratch was measured at the beginning of the experiment and the area of cell migration was quantified after 16 h using ImageJ software. Black bar denotes 200 μM. ( c ) Graph quantifying the area migrated by cells treated with Dox relative to the area migrated by cells treated with vehicle control. For each sample, over 30 non-overlapping fields were measured at each time point; and each experiment was repeated twice. Data are the mean±s.d. ** P <0.001 (Student’s t -test). ( d ) Graph quantifying the distance of outgrowth (μm) of epithelial cells from skin explants from control ( K14-rtTA) or tet-inducible Tcf3 mice ( K14-rtTA;TRE-Tcf3) . Dorsal skin punches (4 mm)were cultured for 8 days in the presence or absence of Dox and proliferation was blocked by mitomycin C treatment on day 3. Explants from a minimum of four mice were analysed for each condition. Data are mean±s.d. ** P <0.01 (Student’s t -test). ( e ) Representative images of epithelial outgrowth from explants that were immunostained with keratin 17 antibody and counterstained with hematoxylin after 8 days in culture. Scale bar, 1 mm. Full size image Tcf3 overexpression promotes cell migration In the re-epithelialization step of the wound repair process, epidermal cells migrate into the wound site, proliferate and differentiate to reform the epidermal barrier [1] . To determine whether Tcf3 is involved in cell migration, we applied an established in vitro cell migration/wounding assay [26] to uncouple cell migration from growth and differentiation effects. In this assay, scratch ‘wounds’ are created in monolayers of mitotically inactivated mouse keratinocytes, and migration of keratinocytes into the scratch is then observed over time. To assess the effect of Tcf3 overexpression on migration, we first performed the assay with primary keratinocytes isolated from tet-inducible Tcf3 ( K14-rtTA;TRE-mycTcf3 ) transgenic mice [22] , which express a tightly regulated, strongly doxycycline (Dox)-inducible Tcf3 transgene under the skin-specific keratin 14 promoter ( Supplementary Fig. 2 ). We found that Tcf3-overexpressing keratinocytes showed an increase in cell migration of 60% compared with non-overexpressing controls (** P <0.001, Student’s t -test) ( Fig. 1b,c ), suggesting that Tcf3 can indeed functionally affect cell migration. Using ex vivo explant skin culture, we also found epithelial cells from Tcf3-induced skins migrated more than the cells from control skins (** P <0.001, Student’s t -test) ( Fig. 1d,e ). To determine whether the ability to promote cell migration is specific to Tcf3 or is a general characteristic of Lef/Tcf family members, we compared the effects of overexpression of all four Lef/Tcf members on cell migration. We transduced keratinocytes with green fluorescent protein (GFP)-tagged, tet-inducible lentiviral vectors [27] carrying myc-tagged Tcf3, Tcf4, Lef1 or Tcf1 transgenes and enriched for transduced cells by fluorescent cell sorting. We then used Dox to induce the expression of the Lef/Tcf genes 24 h prior to performing the migration assay. All four Lef/Tcf members were expressed at similar levels upon Dox treatment ( Supplementary Fig. 3a ). Of the four Lef/Tcf members, only Tcf3 and Tcf4 promoted cell migration (** P <0.001, Student’s t -test) ( Supplementary Fig. 3b,c ). Epidermal Tcf3 overexpression promotes wound healing Since overexpression of Tcf3 promotes cell migration in vitro and ex vivo , we wanted to determine whether Tcf3 expression could promote wound healing in vivo . We created full-thickness, 1 cm × 1 cm wounds on the dorsal skin of tet-inducible Tcf3 ( K14-rtTA;TRE-mycTcf3 ) ( n =5) or control ( K14-rtTA or TRE-mycTcf3 ) ( n =5) mice that had been maintained on a Dox-containing diet. We then measured the surface area of the wounds 6 and 10 days after wounding. We saw that wound closure was significantly accelerated in Tcf3-induced mice relative to controls (* P <0.05, Student’s t -test) ( Fig. 2a,b ). Expression of the Tcf3 transgene was verified by immunofluorescent staining and western for Tcf3 ( Supplementary Fig. 4a,c ). Overexpression of Tcf3 did not lead to an increase in Ki67 staining at the wound edge ( Supplementary Fig. 4b ), suggesting that accelerated wound closure is mainly due to enhanced cell migration and not proliferation. Together with our previous finding that the loss of Tcf3 and Tcf4 causes defective wound repair [23] , our current finding that Tcf3 overexpression is sufficient to promote wound healing strongly suggests a critical role for Tcf3 in normal wound repair in vivo . 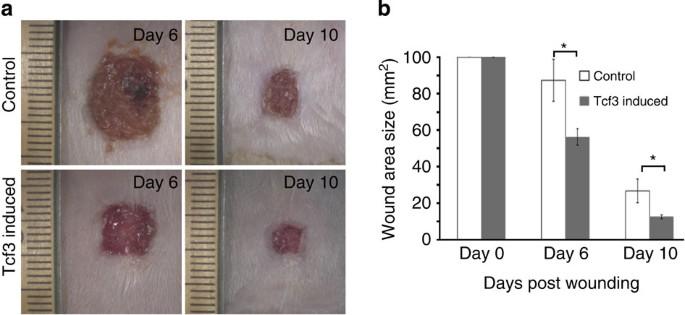Figure 2: Tcf3 overexpression promotes wound healing. (a) Images of skin wound sites taken 6 and 10 days post wounding. An area of 1 cm2full-thickness wounds were created on dorsal skins of tet-inducible Tcf3 (K14-rtTA;TRE-mycTcf3) or control (K14-rtTA or TRE-mycTcf3) mice that had been maintained on a Dox-containing diet (n=5). Six and 10 days after wounding, images of the wound sites were taken and the skins were embedded in OCT for analysis. (b) Graph quantifying the average area of the wounds 6 and 10 days post wounding. Areas of the wounds were measured with ImageJ software. Data are mean±s.d. *P<0.05 (Student’st-test). Figure 2: Tcf3 overexpression promotes wound healing. ( a ) Images of skin wound sites taken 6 and 10 days post wounding. An area of 1 cm 2 full-thickness wounds were created on dorsal skins of tet-inducible Tcf3 ( K14-rtTA;TRE-mycTcf3 ) or control ( K14-rtTA or TRE-mycTcf3 ) mice that had been maintained on a Dox-containing diet ( n =5). Six and 10 days after wounding, images of the wound sites were taken and the skins were embedded in OCT for analysis. ( b ) Graph quantifying the average area of the wounds 6 and 10 days post wounding. Areas of the wounds were measured with ImageJ software. Data are mean±s.d. * P <0.05 (Student’s t -test). Full size image Tcf3 is induced at the wound edge in response to Stat3 Next, we sought to identify factors that regulate Tcf3 expression in response to wounding. We identified three evolutionarily conserved Stat3 binding sites in the Tcf3 promoter ( Supplementary Fig. 5 ), suggesting that Stat3 could potentially activate Tcf3 transcription. Stat3 is one of seven members of the STAT (Signal Transducer and Activator of Transcription) family of transcription factors, which remain latent in the cytoplasm at baseline. Upon activation by phosphorylation on its tyrosine residue 705, Stat3 dimerizes and translocates into the nucleus, where it binds to conserved consensus sites on target genes and activates their transcription [28] . The role of Stat3 in promoting cell migration has been reported in numerous cases [2] , [29] , but the genes directly targeted by Stat3 to regulate cell migration are still largely unknown. Given that Stat3 is induced at the skin wound edge and that its ablation has been shown to impair wound repair [2] , we next examined whether Stat3 regulates Tcf3 expression in response to wounding. As expected, we found activated Stat3 at the wound edge, mirroring the pattern of Tcf3 induction ( Fig. 3a,b ). In contrast, in Stat3 fl/fl ; K14-Cre ( Stat3 cKO) mice, where epidermal Stat3 is conditionally ablated [30] by the epidermis-specific keratin 14 Cre driver [31] , Tcf3 failed to be induced at the skin wound edge ( Fig. 3c,d ). We obtained similar results by in situ hybridization for Tcf3 messenger RNA ( Fig. 3e,f ). Thus, these data suggest that Stat3 is necessary for Tcf3 upregulation during the wound response. Interestingly, Stat3 is not required for the induction of Tcf4 at the wound edge ( Supplementary Fig. 6a ). 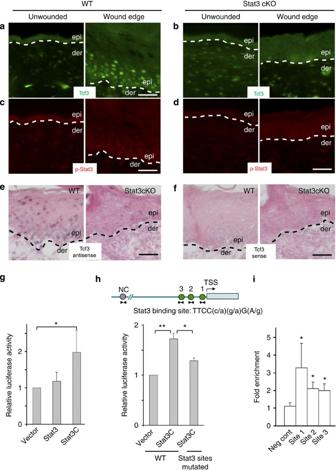Figure 3: Tcf3 induction in response to wounding is dependent on Stat3. (a,b) Full-thickness wounds were created on dorsal skins of 10-week-old mice and isolated 5 days post wounding. Skins containing the wound sites were analysed by immunofluorescence with antibodies against phospho-Y705-Stat3 (red) and Tcf3 (green). Unwounded skins from the same mice were used as controls. Scale bar, 50 μm. (c,d) Images of immunofluorescence analysis of the wound edge of skin fromStat3fl/fl;K14-Cre (Stat3cKO) mice. Unwounded skins from the same mice were used as controls. (e,f)In situhybridization analysis of Tcf3 expression at the wound edge of wild-type andStat3ckO skin using antisense toTcf3as probe (e) compared with Tcf3 sense as a control (f). Scale bar, 50 μm. (g) Keratinocytes were transfected withTcf3promoter-Firefly luciferase andRenillaluciferase constructs, together with constructs expressing either Stat3, constitutively active Stat3 (Stat3C) or control vector. Luciferase activity was measured and Firefly luciferase activity was normalized overRenillaluciferase activity. Graph shows normalized luciferase activity relative to vector control. Experiments were repeated three times. Data are mean±s.d. *P<0.05 (Student’st-test). (h) Schematic showing Stat3 binding sites onTcf3promoter. Keratinocytes were transfected with wild-type or mutatedTcf3promoter–Firefly luciferase andRenillaluciferase constructs, together with constructs expressing Stat3C or empty vector. Graph shows normalized luciferase activity relative to the vector control. Experiments were repeated three times. Data are mean±s.d. *P<0.05, **P<0.01 (Student’st-test). (i) ChIP was performed with anti-Stat3 or isotype control antibodies on cross-linked hair follicle cell chromatin lysate. Amount of chromatin precipitated by Stat3 or IgG was measured by qPCR using primers spanning regions containing Stat3 binding sites (sites 1–3) or regions without Stat3 conserved binding sites (neg cont). The graph shows the amount of fold enrichment of Stat3-immunoprecipitated DNA relative to IgG-immunoprecipitated DNA. Experiments were repeated three times. Data are mean±s.d. *P<0.05 (Student’st-test). Figure 3: Tcf3 induction in response to wounding is dependent on Stat3. ( a , b ) Full-thickness wounds were created on dorsal skins of 10-week-old mice and isolated 5 days post wounding. Skins containing the wound sites were analysed by immunofluorescence with antibodies against phospho-Y705-Stat3 (red) and Tcf3 (green). Unwounded skins from the same mice were used as controls. Scale bar, 50 μm. ( c , d ) Images of immunofluorescence analysis of the wound edge of skin from Stat3 fl/fl ;K14-Cre (Stat3 cKO) mice. Unwounded skins from the same mice were used as controls. ( e , f ) In situ hybridization analysis of Tcf3 expression at the wound edge of wild-type and Stat3 ckO skin using antisense to Tcf3 as probe ( e ) compared with Tcf3 sense as a control ( f ). Scale bar, 50 μm. ( g ) Keratinocytes were transfected with Tcf3 promoter-Firefly luciferase and Renilla luciferase constructs, together with constructs expressing either Stat3, constitutively active Stat3 (Stat3C) or control vector. Luciferase activity was measured and Firefly luciferase activity was normalized over Renilla luciferase activity. Graph shows normalized luciferase activity relative to vector control. Experiments were repeated three times. Data are mean±s.d. * P <0.05 (Student’s t -test). ( h ) Schematic showing Stat3 binding sites on Tcf3 promoter. Keratinocytes were transfected with wild-type or mutated Tcf3 promoter–Firefly luciferase and Renilla luciferase constructs, together with constructs expressing Stat3C or empty vector. Graph shows normalized luciferase activity relative to the vector control. Experiments were repeated three times. Data are mean±s.d. * P <0.05, ** P <0.01 (Student’s t -test). ( i ) ChIP was performed with anti-Stat3 or isotype control antibodies on cross-linked hair follicle cell chromatin lysate. Amount of chromatin precipitated by Stat3 or IgG was measured by qPCR using primers spanning regions containing Stat3 binding sites (sites 1–3) or regions without Stat3 conserved binding sites (neg cont). The graph shows the amount of fold enrichment of Stat3-immunoprecipitated DNA relative to IgG-immunoprecipitated DNA. Experiments were repeated three times. Data are mean±s.d. * P <0.05 (Student’s t -test). Full size image We next tested Stat3-mediated Tcf3 promoter activation by luciferase reporter assays, using a 5 kb Tcf3 promoter fragment cloned from genomic DNA. We found that constitutively activated Stat3 (Stat3C) induced reporter expression from the Tcf3 promoter; activation of the reporter was abolished by mutation of the Stat3 binding sites (* P <0.05, Student’s t -test) ( Fig. 3g,h ). Lef1 and Tcf1 do not contain conserved Stat3 binding sites in their promoters while Tcf4 contains one conserved Stat3 binding site. However, Stat3C did not induce reporter expression from the 5 kb Tcf4 promoter in the luciferase reporter assay ( Supplementary Fig. 6b ). To determine whether endogenous Stat3 directly binds to the Tcf3 promoter in vivo , we used an antibody against Stat3 to perform chromatin immunoprecipitation (ChIP) on chromatin lysates from hair follicle cells where phosphorylated Stat3 was detectable by western analysis (data not shown). We detected endogenous Stat3 bound to the Tcf3 promoter in regions containing conserved Stat3 binding sites (* P <0.05, Student’s t -test), but not in control regions that lack Stat3 binding sites ( Fig. 3i ). ChIP on chromatin lysates from wounded skins also showed Stat3 binding to the Tcf3 promoter ( Supplementary Fig. 7 ). These results suggest that Stat3 directly binds and activates the Tcf3 promoter. Although Stat3 activates the Tcf3 promoter in vitro and binds to the endogenous Tcf3 promoter in vivo , overexpression of constitutively activated Stat3 (Stat3C) in the epidermis was not sufficient to induce expression of Tcf3 ( Supplementary Fig. 8a,b ). Furthermore, ablation of Stat3 in the skin does not alter the expression pattern of Tcf3 during normal development and homeostasis, as Tcf3 is expressed at similar levels in Stat3-deficient skin compared with wild-type skin ( Supplementary Fig. 8c,d ). Thus, although it is required for upregulation of Tcf3 in response to wounding, Stat3 activation alone is insufficient to activate Tcf3 expression. Tcf3 rescues defective migration in Stat3-deficient cells Previous reports have shown that ablation of epidermal Stat3 impairs cutaneous wound repair in vivo and cell migration in vitro [2] . Given our observations that Stat3 is required for Tcf3 induction at the skin wound edge and that Tcf3 promotes cell migration, the promotion of cell migration by Stat3 might be dependent on its induction of Tcf3. To address this, we next determined whether Tcf3 overexpression could rescue the cell migration defect caused by deficiency of Stat3. We cultured primary keratinocytes from Stat3 fl/fl ;K14-Cre (Stat3 cKO) mice [30] , transduced them with GFP-tagged lentiviral vectors expressing tet-inducible Tcf3, and enriched them by fluorescent cell sorting. We then treated the cells with Dox to induce expression of Tcf3 just prior to the migration assay. As expected, Stat3 cKO keratinocytes showed impaired cell migration (** P <0.001, Student’s t -test). Importantly, this defect was reversed by Tcf3 overexpression (** P <0.001, Student’s t -test) ( Fig. 4a,b ). The observation that transgenically induced Tcf3 can rescue defective migration in Stat3-deficient keratinocytes strongly suggests that Tcf3 is a key downstream effector of Stat3 in this process. 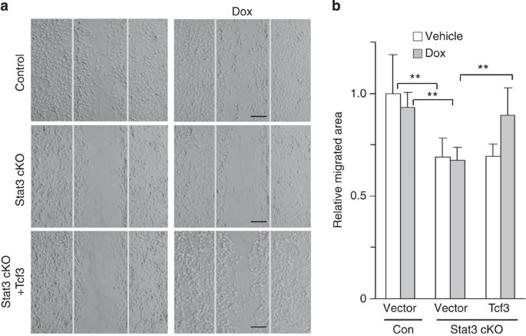Figure 4: Tcf3 induction rescues the defective migration in Stat3-deficient cells. (a) Primary keratinocytes fromStat3fl/fl(cont) orStat3fl/fl;K14-Cre (Stat3cKO) mice were isolated and were transduced with GFP-tagged lentiviral vector expressing tet-inducible Tcf3 or with empty vector control. After the transduced cells were enriched by fluorescent cell sorting, they were grown to confluence and then subjected to a migration assay with or without Dox. Images of keratinocytes 48 h after initiation of the migration assay. Black bar denotes 200 μm. (b) Graph quantifying the relative area the cells migrated normalized over vehicle control. For each sample, over 30 non-overlapping fields were measured at each time point; and each experiment was repeated three times. Data are the mean±s.d. **P<0.001 (Student’st-test). Figure 4: Tcf3 induction rescues the defective migration in Stat3-deficient cells. ( a ) Primary keratinocytes from Stat3 fl/fl (cont) or Stat3 fl/fl ; K14-Cre (Stat3 cKO) mice were isolated and were transduced with GFP-tagged lentiviral vector expressing tet-inducible Tcf3 or with empty vector control. After the transduced cells were enriched by fluorescent cell sorting, they were grown to confluence and then subjected to a migration assay with or without Dox. Images of keratinocytes 48 h after initiation of the migration assay. Black bar denotes 200 μm. ( b ) Graph quantifying the relative area the cells migrated normalized over vehicle control. For each sample, over 30 non-overlapping fields were measured at each time point; and each experiment was repeated three times. Data are the mean±s.d. ** P <0.001 (Student’s t -test). Full size image Tcf3 promotes cell migration independently of β-catenin In light of the important role of Tcf3 in cell migration and wound healing, we sought to identify the mechanism by which Tcf3 affect this process. Since Tcf3 can function as both a β-catenin-dependent transcriptional activator and a β-catenin-independent repressor, we first tested which of these functions is necessary in cell migration. We transduced keratinocytes with GFP-tagged, tet-inducible lentiviral vectors carrying either myc-tagged wild-type Tcf3 or one of two Tcf3 deletion mutants: Tcf3ΔN, which does not bind to β-catenin and therefore cannot activate Wnt target genes; and Tcf3ΔG, which cannot bind Groucho/TLE-family corepressors and thus loses repressor function [20] . After enrichment by fluorescent cell sorting, the transduced cells were treated with Dox to induce the expression of wild-type or mutant Tcf3 ( Fig. 5a ; Supplementary Fig. 9a ), and then subjected to the in vitro wounding assay. We found that overexpressing Tcf3ΔN promoted cell migration to a similar extent as wild-type Tcf3 (** P <0.001, Student’s t -test), while overexpressing Tcf3ΔG produced no significant effect on migration ( Fig. 5b,c ). We therefore conclude that the promigratory effect of Tcf3 does not require its β-catenin-interacting domain but depends on its repressor function. However, we should note that although the loss of pro-migratory effect of Tcf3ΔG correlates with its loss of repressor function, we cannot definitively claim it is due to its loss of interaction with Groucho per se , since the ΔG mutation also affects binding to proteins other than Groucho corepressors. 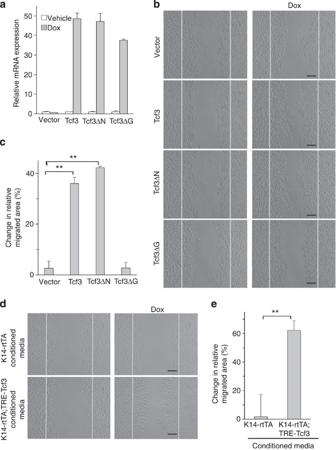Figure 5: Tcf3 promotes cell migration non-cell autonomously and independently of its role as a cofactor to β-catenin. (a) Real-time PCR analysis of level of expression of transduced tet-inducible Tcf3 and its mutant versions, Tcf3ΔN and Tcf3ΔG, in response to Dox. Keratinocytes were transduced with GFP-tagged, tet-inducible lentivectors carrying myc-tagged Tcf3 or its mutant versions. Transduced cells were isolated by fluorescent cell sorting and were treated with Dox or vehicle control for 24 h prior to being harvested for messenger RNA analysis. Mean expression values from biological duplicates were calculated. Data are mean±s.d. (Student’st-test). (b) Images of transduced keratinocytes expressing tet-inducible Tcf3, Tcf3ΔN, Tcf3ΔG 16 h after the initiation of migration assay with or without Dox. Black bar denotes 200 μm. (c) Graph quantifying the area migrated by transduced cells treated with Dox relative to the area migrated by cells treated with vehicle control. For each sample, over 30 non-overlapping fields were measured at each time point; and each experiment was repeated twice. Data are mean±s.d. **P<0.001 (Student’st-test). (d) Tcf3-induced cells secrete factors that promote cell migration. Keratinocytes from tet-inducible Tcf3 (K14-rtTA;TRE-mycTcf3)and control(K14-rtTA)mice were cultured in the presence or absence of Dox for 48 h and their conditioned media were collected. Wild-type keratinocytes were subjected to a migration assay in the presence of specified conditioned media. Images were taken 38 h after the initiation of migration assay. Scale bar, 200 μm. (e) Conditioned media from Tcf3-induced cells (K14-rtTA;TRE-mycTcf3+Dox) promotes migration of wild-type cells. Graph quantifying the migrated area of wild-type cells that were incubated with Dox-treated conditioned media during the migration assay relative to the area migrated by cells treated with vehicle-treated conditioned media. For each sample, over 30 non-overlapping fields were measured at each time point; and each experiment was repeated three times. Data are mean±s.d. **P<0.001 (Student’st-test). Figure 5: Tcf3 promotes cell migration non-cell autonomously and independently of its role as a cofactor to β-catenin. ( a ) Real-time PCR analysis of level of expression of transduced tet-inducible Tcf3 and its mutant versions, Tcf3ΔN and Tcf3ΔG, in response to Dox. Keratinocytes were transduced with GFP-tagged, tet-inducible lentivectors carrying myc-tagged Tcf3 or its mutant versions. Transduced cells were isolated by fluorescent cell sorting and were treated with Dox or vehicle control for 24 h prior to being harvested for messenger RNA analysis. Mean expression values from biological duplicates were calculated. Data are mean±s.d. (Student’s t -test). ( b ) Images of transduced keratinocytes expressing tet-inducible Tcf3, Tcf3ΔN, Tcf3ΔG 16 h after the initiation of migration assay with or without Dox. Black bar denotes 200 μm. ( c ) Graph quantifying the area migrated by transduced cells treated with Dox relative to the area migrated by cells treated with vehicle control. For each sample, over 30 non-overlapping fields were measured at each time point; and each experiment was repeated twice. Data are mean±s.d. ** P <0.001 (Student’s t -test). ( d ) Tcf3-induced cells secrete factors that promote cell migration. Keratinocytes from tet-inducible Tcf3 ( K14-rtTA;TRE-mycTcf3) and control (K14-rtTA) mice were cultured in the presence or absence of Dox for 48 h and their conditioned media were collected. Wild-type keratinocytes were subjected to a migration assay in the presence of specified conditioned media. Images were taken 38 h after the initiation of migration assay. Scale bar, 200 μm. ( e ) Conditioned media from Tcf3-induced cells ( K14-rtTA;TRE-mycTcf3 +Dox) promotes migration of wild-type cells. Graph quantifying the migrated area of wild-type cells that were incubated with Dox-treated conditioned media during the migration assay relative to the area migrated by cells treated with vehicle-treated conditioned media. For each sample, over 30 non-overlapping fields were measured at each time point; and each experiment was repeated three times. Data are mean±s.d. ** P <0.001 (Student’s t -test). Full size image Tcf3 promotes cell migration non-cell autonomously We next determined whether Tcf3 promotes cell migration cell autonomously or by paracrine effects on neighbouring cells. We cultured tet-inducible Tcf3 keratinocytes ( K14-rtTA;TRE-mycTcf3 ) or single transgenic controls ( K14-rtTA ) in the presence or absence of Dox and collected their conditioned media (CM). We then tested the ability of the CM to influence migration of wild-type keratinocytes. Cells that were incubated with CM from Tcf3-overexpressing cells displayed enhanced migration compared with cells incubated with control CM (** P <0.001, Student’s t -test). This suggests that Tcf3-induced cells produce secreted factors that affect the migration of wild-type cells ( Fig. 5d,e ) and implies that Tcf3 promotes cell migration non-cell autonomously. Moreover, we found that CM from Tcf3ΔN-, but not Tcf3ΔG-overexpressing cells promoted cell migration (** P <00.1, Student’s t -test), confirming that indeed Tcf3 promotes cell migration independently of β-catenin and non-cell autonomously ( Supplementary Fig. 9b ). Since Tcf3 promotes cell migration non-cell autonomously, we wanted to determine whether Tcf3 also non-cell autonomously promotes wound healing. After creating full thickness wounds of 1 cm 2 on the dorsal skin of wild-type mice, we applied concentrated CM from Tcf3-overexpressing cells (Tcf3-CM) or control cells onto the wound sites ( n =5 each group). We found that daily application of Tcf3-CM onto the wound sites significantly accelerated wound closure (* P <0.05, Student’s t -test) ( Fig. 6a,b ). 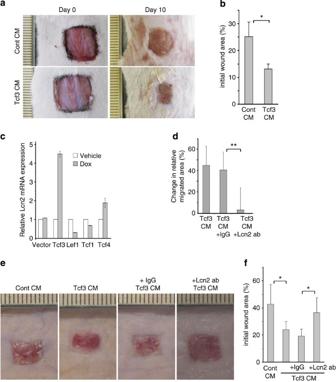Figure 6: Lcn2 is the key secreted mediator of Tcf3-induced cell migration and wound healing. (a) Images of skin wound sites taken immediately after wounding and 10 days post wounding. After full-thickness wounds of 1 cm2were created on the dorsal skins of wild-type mice (n=5), CM from Tcf3-overexpressing cells or control cells was applied topically onto the wound sites daily for a week. Surface areas of the wounds were measured at the initial time point and 10 days post wounding. (b) Graph quantifying the surface areas of the wounds as a percentage of the original wounds 10 days post wounding. Data are mean±s.d. *P<0.05 (Student’st-test). (c) Real-time PCR analysis of Lcn2 expression in keratinocytes that were transduced to express tet-inducible Lef/Tcf members. Keratinocytes were transduced with GFP-tagged, tet-inducible lentivectors carrying myc-tagged Lef/Tcf members. Transduced cells were isolated by FACS (fluorescence-activated cell sorting) and were treated with Dox or vehicle control for 24 h prior to being harvested for messenger RNA analysis. Mean expression values from biological triplicates were calculated. Data are mean±s.d. (d) Migration assays were performed on keratinocytes that were incubated with control CM or Tcf3-CM together with anti-Lcn2 antibody or IgG isotype control. Graph quantifying the relative area migrated by keratinocytes treated with Tcf3-CM incubated with IgG or anti-Lcn2 normalized over area migrated by cells treated with control CM. For each sample, over 30 non-overlapping fields were measured at each time point; and each experiment was repeated twice. Data are mean±s.d. **P<0.001 (Student’st-test). (e) Images of the wound sites were taken 10 days post wounding. 1 cm2full-thickness wounds were created on dorsal skins ofnudemice and were treated daily with topical application of conditioned media from control (empty vector) CM (cont-CM) or Tcf3-CM untreated or pre-incubated with antibodies against Lcn2 or isotype control. (f) Graph quantifying the surface areas of the wounds as a percentage of the original wounds 10 days post wounding, cont-CM (n=7) or Tcf3-CM untreated (n=7) or preincubated with antibodies against Lcn2 (n=8) or isotype control (n=6). Surface areas of the wounds were measured at the initial time point and 10 days post wounding. Data are mean±s.d. *P<0.05 (Student’st-test). Figure 6: Lcn2 is the key secreted mediator of Tcf3-induced cell migration and wound healing. ( a ) Images of skin wound sites taken immediately after wounding and 10 days post wounding. After full-thickness wounds of 1 cm 2 were created on the dorsal skins of wild-type mice ( n =5), CM from Tcf3-overexpressing cells or control cells was applied topically onto the wound sites daily for a week. Surface areas of the wounds were measured at the initial time point and 10 days post wounding. ( b ) Graph quantifying the surface areas of the wounds as a percentage of the original wounds 10 days post wounding. Data are mean±s.d. * P <0.05 (Student’s t -test). ( c ) Real-time PCR analysis of Lcn2 expression in keratinocytes that were transduced to express tet-inducible Lef/Tcf members. Keratinocytes were transduced with GFP-tagged, tet-inducible lentivectors carrying myc-tagged Lef/Tcf members. Transduced cells were isolated by FACS (fluorescence-activated cell sorting) and were treated with Dox or vehicle control for 24 h prior to being harvested for messenger RNA analysis. Mean expression values from biological triplicates were calculated. Data are mean±s.d. ( d ) Migration assays were performed on keratinocytes that were incubated with control CM or Tcf3-CM together with anti-Lcn2 antibody or IgG isotype control. Graph quantifying the relative area migrated by keratinocytes treated with Tcf3-CM incubated with IgG or anti-Lcn2 normalized over area migrated by cells treated with control CM. For each sample, over 30 non-overlapping fields were measured at each time point; and each experiment was repeated twice. Data are mean±s.d. ** P <0.001 (Student’s t -test). ( e ) Images of the wound sites were taken 10 days post wounding. 1 cm 2 full-thickness wounds were created on dorsal skins of nude mice and were treated daily with topical application of conditioned media from control (empty vector) CM (cont-CM) or Tcf3-CM untreated or pre-incubated with antibodies against Lcn2 or isotype control. ( f ) Graph quantifying the surface areas of the wounds as a percentage of the original wounds 10 days post wounding, cont-CM ( n =7) or Tcf3-CM untreated ( n =7) or preincubated with antibodies against Lcn2 ( n =8) or isotype control ( n =6). Surface areas of the wounds were measured at the initial time point and 10 days post wounding. Data are mean±s.d. * P <0.05 (Student’s t -test). Full size image Lcn2 is the key mediator of Tcf3 in wound healing Since Tcf3 promotes cell migration and wound healing in a non-cell autonomous manner, we sought to identify the secreted factors involved in this process. We searched previously compiled microarray data for genes encoding extracellular proteins that were upregulated upon Tcf3 overexpression [22] . Of the potential candidates, we focused on lipocalin2 (Lcn2, also known as NGAL, 24p3, uterocalin or siderocalin) since it has been reported to play a role in promoting cell motility in both neurons and cancer cells [32] , [33] , [34] , [35] . It has also been shown to stimulate colonic cell migration and gut tissue repair [36] . Lcn2 is an acute-phase protein expressed in certain tissues in response to injury and inflammation [37] . It is also overexpressed in many types of cancer and has been implicated in metastasis in breast cancer [32] , [38] , [39] . We verified that Lcn2 expression is increased in response to Tcf3 overexpression in both cultured keratinocytes ( Fig. 6c and Supplementary Fig. 10a,b ) and in vivo in skin ( Supplementary Fig. 10c ). We also found that Lcn2 expression is induced at the wound edge ( Supplementary Fig. 10d,e ). To determine whether Tcf3 promotes cell migration and wound healing through upregulation of Lcn2, we incubated the CM collected from Tcf3 overexpressing cells (Tcf3-CM) with antibodies against Lcn2 and evaluated how the inhibition of Lcn2 affects cell migration and wound healing. We found that immunodepletion of Lcn2 from Tcf3-CM reversed the promigratory effect in vitro (** P <0.001, Student’s t -test) ( Fig. 6d ) and its prowound closure effect in vivo (* P <0.05, Student’s t -test) ( Fig. 6e,f ). A similar loss of efficacy was observed following Lcn2 immunodepletion in the ex vivo explant culture system (* P <0.05, Student’s t -test) ( Supplementary Fig. 11 ). We also found that Tcf3-CM collected from Lcn2 KO cells did not promote wound closure in contrast to the Tcf3-CM collected from WT cells (** P <0.001, Student’s t -test) ( Supplementary Fig. 12 ). Together, these results suggest that Tcf3 promotes cell migration and wound healing through upregulation of the secreted factor Lcn2. Since our data suggest that the promigratory effects of Tcf3 are dependent on its transcriptional repressor function, the induction of Lcn2 due to Tcf3 overexpression is most likely an indirect effect. To determine whether Lcn2 alone is sufficient to promote epidermal cell migration, we tested the effect of CM collected from Lcn2-overexpressing cells (Lcn2-CM) on cell migration. We found that keratinocytes that were incubated in Lcn2-CM migrated more than keratinocytes incubated with control CM (** P <0.001, Student’s t -test) ( Fig. 7a ). To determine whether Lcn2 itself can promote wound healing in vivo , we topically applied Lcn2-CM onto full-thickness wounds and evaluated its effect on the wound repair process. We found that the application of Lcn2-CM ( n =4) accelerated wound closure significantly (* P <0.05, Student’s t -test) more than the application of control CM ( n =4) ( Fig. 7b,c ). Similarly, the application of recombinant Lcn2 protein onto wounds also substantially accelerated wound closure ( n =6) (* P <0.05, Student’s t -test) ( Supplementary Fig. 13 ). Since overexpression of Lcn2 does not promote proliferation in vitro ( Supplementary Fig. 10f ), these data suggest that Lcn2 promotes wound healing by promoting cell migration. 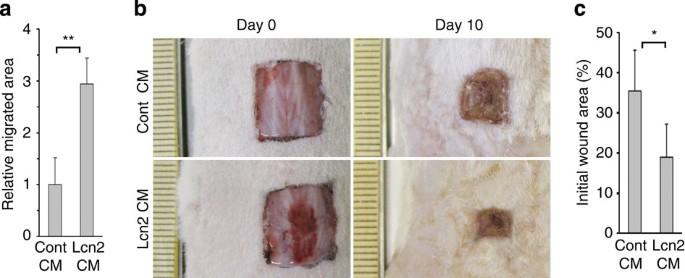Figure 7: Lcn2 is sufficient to promote cell migration and wound healing. (a) Migration assays were performed on keratinocytes that were incubated with Lcn2-CM or control (empty vector) CM (cont). Graph quantifying the relative migrated area of keratinocytes treated with the indicated CM. For each sample, over 30 non-overlapping fields were measured at each time point; and each experiment was repeated twice. Data are mean±s.d. **P<0.001. (b) Full-thickness wounds (1 cm2) were created on dorsal skins of wild-type mice (n=4) and were treated daily with topical application of conditioned media (CM) from Lcn2 (n=4) or control (empty vector) (n=5) transduced keratinocytes. Images of the wound sites were taken at the beginning of the wounding experiment and 10 days post wounding, at which point skins were harvested for analysis. (c) Graph quantifying the effect of topical application of Lcn2-CM on wound closure, conditioned media (CM) from Lcn2 (n=4) or control (empty vector) (n=5). Average surface areas of the wounds 10 days post wounding is quantified as a percentage of the initial wound areas. Areas of the wounds were measured with ImageJ software. Data are mean±s.d. *P<0.05 (Student’st-test). Figure 7: Lcn2 is sufficient to promote cell migration and wound healing. ( a ) Migration assays were performed on keratinocytes that were incubated with Lcn2-CM or control (empty vector) CM (cont). Graph quantifying the relative migrated area of keratinocytes treated with the indicated CM. For each sample, over 30 non-overlapping fields were measured at each time point; and each experiment was repeated twice. Data are mean±s.d. ** P <0.001. ( b ) Full-thickness wounds (1 cm 2 ) were created on dorsal skins of wild-type mice ( n =4) and were treated daily with topical application of conditioned media (CM) from Lcn2 ( n =4) or control (empty vector) ( n =5) transduced keratinocytes. Images of the wound sites were taken at the beginning of the wounding experiment and 10 days post wounding, at which point skins were harvested for analysis. ( c ) Graph quantifying the effect of topical application of Lcn2-CM on wound closure, conditioned media (CM) from Lcn2 ( n =4) or control (empty vector) ( n =5). Average surface areas of the wounds 10 days post wounding is quantified as a percentage of the initial wound areas. Areas of the wounds were measured with ImageJ software. Data are mean±s.d. * P <0.05 (Student’s t -test). Full size image To determine whether Lcn2 is essential in the wound repair process, we immunodepleted Lcn2 by topically applying anti-Lcn2 ( n =8) or isotype control antibodies ( n =8) onto full-thickness wounds in nude mice. Wounds that were treated with the Lcn2 blocking antibody repaired less efficiently than the wounds that were treated with immunoglobulin G (IgG) control (* P <0.05, Student’s t -test) ( Fig. 8a,b ). More importantly, we also found that Lcn2 KO mice repaired their wounds less efficiently than WT mice ( n =7) (** P <0.001, Student’s t -test) ( Fig. 8c,d ). These data demonstrate that Lcn2 is required for efficient wound repair. 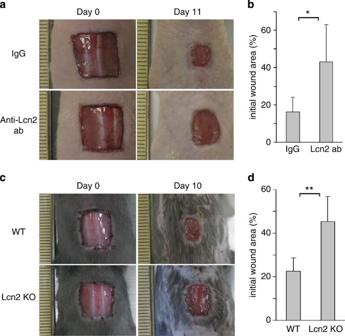Figure 8: Lipocalin2 is required for efficient wound healing. (a) Images of skin wound sites taken immediately after wounding and 11 days post wounding. After full-thickness wounds of 1 cm2were created on the dorsal skins ofnudemice, anti-Lcn2 (n=8) or isotype control (n=6) antibodies were applied topically onto the wound sites every other day. Surface areas of the wounds were measured at the initial time point and 11 days post wounding. (b) Graph quantifying the surface areas of the wounds as a percentage of the original wounds 11 days post wounding, anti-Lcn2 (n=8) or isotype control (n=6). Data are mean±s.d. *P<0.05 (Student’st-test). (c) Images of skin wound sites taken immediately after wounding and 10 days post wounding of WT andLcn2KO mice. Wounds 1 cm2were created on the dorsal skins of WT andLcn2KO mice (n=7). Surface areas of the wounds were measured at the initial time point and 10 days post wounding. (d) Graph quantifying the surface areas of the wounds as a percentage of the original wounds 10 days post wounding, WT (n=7) andLcn2KO mice (n=7). Data are mean±s.d. **P<0.001 (Student’st-test). Figure 8: Lipocalin2 is required for efficient wound healing. ( a ) Images of skin wound sites taken immediately after wounding and 11 days post wounding. After full-thickness wounds of 1 cm 2 were created on the dorsal skins of nude mice, anti-Lcn2 ( n =8) or isotype control ( n =6) antibodies were applied topically onto the wound sites every other day. Surface areas of the wounds were measured at the initial time point and 11 days post wounding. ( b ) Graph quantifying the surface areas of the wounds as a percentage of the original wounds 11 days post wounding, anti-Lcn2 ( n =8) or isotype control ( n =6). Data are mean±s.d. * P <0.05 (Student’s t -test). ( c ) Images of skin wound sites taken immediately after wounding and 10 days post wounding of WT and Lcn2 KO mice. Wounds 1 cm 2 were created on the dorsal skins of WT and Lcn2 KO mice ( n =7). Surface areas of the wounds were measured at the initial time point and 10 days post wounding. ( d ) Graph quantifying the surface areas of the wounds as a percentage of the original wounds 10 days post wounding, WT ( n =7) and Lcn2 KO mice ( n =7). Data are mean±s.d. ** P <0.001 (Student’s t -test). Full size image Lcn2 rescues defective migration in Stat3-deficient cells Since Tcf3 overexpression can rescue defective cell migration in Stat3-deficient keratinocytes and Lcn2 is the key mediator of the Tcf3-induced promigratory effect, we sought to determine whether inhibition of Lcn2 could compromise the Tcf3-mediated rescue of Stat3-deficient keratinocytes. We first transduced primary keratinocytes from Stat3 fl/fl ;K14-Cre (Stat3 cKO) mice with a GFP-tagged lentiviral vector expressing tet-inducible Tcf3 or an empty vector control. After enriching them by fluorescent cell sorting, we then treated the cells with Dox to induce expression of Tcf3 prior to the migration assay. At the start of the migration assay, we added the Lcn2 blocking antibody or isotype control antibody to the keratinocytes and then quantified the migrated area after 48 h. As in our previous experiments, Stat3-deficient keratinocytes migrated less than the control ( K14-cre ; Stat3 +/ fl ) keratinocytes and overexpression of Tcf3 reversed this migration defect. However, when Lcn2 was depleted, overexpression of Tcf3 could no longer rescue the defective migration in Stat3-deficient keratinocytes (** P <0.001, Student’s t -test) ( Fig. 9a , Supplementary Fig. 14 ). 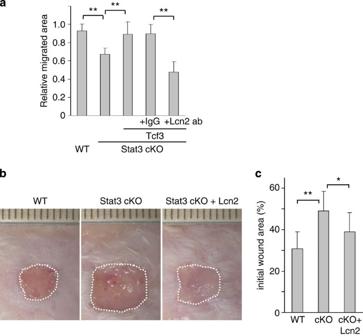Figure 9: Lipocalin2 can rescue defective wound healing inStat3cKO mice. (a) Migration assays were performed onStat3+/fl:K14-cre(cont) orStat3fl/fl:K14-cre(Stat3cKO) keratinocytes that were transduced with control or tet-inducible Tcf3 treated with Dox together with anti-Lcn2 antibody or IgG isotype control. Graph quantifying the relative area migrated by keratinocytes normalized over area migrated by cells transduced with control vector without Dox. For each sample, over 30 non-overlapping fields were measured at each time point; and each experiment was repeated twice. Data are mean±s.d. **P<0.001 (Student’st-test). (b) Images of skin wound sites taken 10 days post wounding. After full-thickness wounds of 1 cm2were created on the dorsal skins of wild-type andStat3cKO mice, 200 μl of recombinant Lcn2 (2 μg ml−1) or vehicle were applied topically onto the wound sites every other day. Surface areas of the wounds were measured at the initial time point and 10 days post wounding. (c) Graph quantifying the surface areas of the wounds as a percentage of the original wounds 10 days post wounding. Wild type (n=13) andStat3cKO (n=7). Data are mean±s.d. *P<0.05 and **P<0.001 (Student’st-test). Figure 9: Lipocalin2 can rescue defective wound healing in Stat3 cKO mice. ( a ) Migration assays were performed on Stat3 +/fl : K14-cre (cont) or Stat3 fl/fl : K14-cre ( Stat3 cKO) keratinocytes that were transduced with control or tet-inducible Tcf3 treated with Dox together with anti-Lcn2 antibody or IgG isotype control. Graph quantifying the relative area migrated by keratinocytes normalized over area migrated by cells transduced with control vector without Dox. For each sample, over 30 non-overlapping fields were measured at each time point; and each experiment was repeated twice. Data are mean±s.d. ** P <0.001 (Student’s t -test). ( b ) Images of skin wound sites taken 10 days post wounding. After full-thickness wounds of 1 cm 2 were created on the dorsal skins of wild-type and Stat3 cKO mice, 200 μl of recombinant Lcn2 (2 μg ml −1 ) or vehicle were applied topically onto the wound sites every other day. Surface areas of the wounds were measured at the initial time point and 10 days post wounding. ( c ) Graph quantifying the surface areas of the wounds as a percentage of the original wounds 10 days post wounding. Wild type ( n =13) and Stat3 cKO ( n =7). Data are mean±s.d. * P <0.05 and ** P <0.001 (Student’s t -test). Full size image Lcn2 rescues defective wound repair in Stat3-deficient skin We next examined whether Lcn2 expression could rescue the defective wound repair process in Stat3-deficient skin. We created full-thickness wounds on Stat3 cKO ( n =11) or control mice ( n =13) and applied recombinant Lcn2 protein or vehicle control onto the wound beds. As expected, Stat3 cKO skin showed defective wound repair (** P <0.001, Student’s t -test). Importantly, the application of recombinant Lcn2 partially rescued the defective wound healing in Stat3 cKO skin (* P <0.05, Student’s t -test) ( Fig. 9b,c ). These data suggest that Stat3’s role in cell migration and wound healing is mediated in part by Lcn2 via Tcf3. To understand and enhance the wound repair process, it is essential to understand the molecular mechanisms underlying the steps contributing to wound repair. Stat3 is one of the few known transcription factors that have been implicated in cell migration and re-epithelialization during wound repair. Conditional ablation of Stat3 in the mammalian epidermis impairs cutaneous wound healing in vivo and epidermal cell migration in vitro [2] . Stat3 deficiency causes cell migration defects during gastrulation in zebrafish [29] . Mice carrying null alleles of Stat3 also die during early gastrulation [40] , suggesting that Stat3 plays a similar role in cell migration during mouse development. In addition, aberrant Stat3 activity promotes tumour invasion and metastasis in various cancers [41] , [42] , [43] , [44] , [45] . Despite the evident role of Stat3 in cell migration, the downstream genes targeted by Stat3 to regulate cell migration are still largely unknown. Our demonstration that Stat3 directly upregulates Tcf3 expression during wounding and that Stat3 can directly activate Tcf3 transcription provides the first direct link between the Stat3 and Tcf3 transcriptional networks, both of which are crucial for tissue homeostasis. More importantly, we show that Tcf3 itself promotes cell migration and that its forced expression rescues defective cell migration in Stat3-deficient cells. Our data not only uncover a novel role for Tcf3 in cell migration, they also suggest that Stat3 promotes cell migration through upregulation of Tcf3. Moreover, our findings that Tcf3 is induced in response to wounding and directly promotes wound healing demonstrate a crucial role for transcriptional regulation of Lef/Tcf factors in determining functional outcomes. This is in contrast with the traditional model in which Tcf activity is primarily regulated by the presence or absence of nuclear β-catenin. In addition, our finding that Tcf3 can promote cell migration without its β-catenin-interacting domain presents a novel β-catenin-independent role for Tcf3 and underlines the importance of Tcf3’s ability to act as a transcriptional repressor. It is interesting to note that overexpression a ΔNLef, a truncated Lef1 that lacks a β-catenin binding site, in the skin results in a delay of wound closure [46] . Because ΔNLef inhibits β-catenin signalling, it is thought that impaired Wnt signalling may be the cause of the delay in wound healing. Indeed, normal proliferation of the interfollicular epidermis requires β-catenin [47] , [48] , and topical application of Wnt3a can accelerate wound repair in the ear wound model [49] . However, inhibition of Wnt signalling by overexpression of the Wnt inhibitor Dkk1 does not alter dorsal skin wound closure, instead affecting only hair follicle neogenesis [50] . Conversely, overexpression of Wnt (Wnt7a) also does not affect dorsal skin wound closure [50] . Although we observed that Tcf3 does not require its β-catenin-interacting domain to promote cell migration in vitro , we cannot currently rule out that in vivo Tcf3 might have a β-catenin-dependent role in wound repair. Finally, our novel observation that Tcf3 acts non-cell-autonomously via Lcn2 to promote migration and wound healing offers a new mechanism by which Tcf3 acts to shape the tissue microenvironment during wounding. We have shown that topical application of CM collected from Tcf3-overexpressing cells or Lcn2-overexpressing cells both enhance wound healing in mice. Blockade of Lcn2 impairs wound healing and diminishes Tcf3-CM’s ability to affect cell migration, suggesting that the secretion of Lcn2 is both necessary and sufficient to promote cell migration and wound healing in response to Tcf3. Lcn2 is an acute phase protein, upregulated at sites of inflammation and injury [33] , [37] , [51] . It is an established biomarker for renal injury, and its levels are increased in serum of patients with psoriasis [52] , [53] . It is also expressed at a high level in a variety of tumours [54] , [55] , [56] , [57] . Lcn2’s diverse roles range from being a bacteriostatic agent to a promoter of cell motility [36] , [58] , [59] . Lcn2’s role in cell migration has been shown in several model systems. Ablation of Lcn2 results in impaired migration of astrocytes to injury sites in both mice and zebrafish [35] , [60] . Overexpression of Lcn2 in vitro increases cell motility and invasiveness of breast cancer cells [32] , [33] . Although Lcn2 can promote cell motility, the molecular mechanism underlying this function is not known. Overexpression of Lcn2 downregulates expression of E-cadherin and increases expression of mesenchymal markers, while downregulation of Lcn2 inhibits cell migration and the mesenchymal phenotype [33] . Based on this finding, it is conceivable that Lcn2 promotes cell migration by affecting cell adhesion via its downregulation of E-cadherin. However, how Lcn2 brings about the downregulation of E-cadherin is still unknown. Furthermore, since Lcn2 binds to and stabilizes matrix metalloproteinase-9 (ref. 61 ), a proteinase that is important for cell migration and wound healing, it is also possible that Lcn2 promotes cell migration by increasing the activity of MMP-9. MMP-9 belongs to the MMP family of zinc-dependent endopeptidases that degrade components of the extracellular matrix, allowing cell migration to occur [62] . Mice with MMP-9 deficiency show delayed cell migration and wound repair [63] . Although it remains to be elucidated how Lcn2 promotes cell migration, our findings clearly demonstrate that Lcn2 has a crucial role in promoting epidermal cell migration and wound healing in skin. We show that the application of Lcn2 to the wound sites substantially accelerates wound healing while the application of antibodies against Lcn2 significantly delays wound healing. Importantly, we also show Lcn2 deficiency results in retarded wound repair. In addition, the application of Lcn2 partially rescues defective wound healing in Stat3-deficient skin, suggesting that Stat3 acts through Tcf3’s downstream effector Lcn2. Although our data clearly show that Tcf3 overexpression induces the expression of Lcn2 and promotes cell migration and wound healing, we still do not know how Tcf3 brings about the induction of Lcn2. Tcf3’s promotion of cell migration is dependent on its ability to act as a repressor and not as an activator. Hence, it is likely that Tcf3 represses repressor(s) of Lcn2 expression, which consequently leads to the induction of Lcn2. We are currently seeking to identify the regulator(s) of Lcn2 that Tcf3 affects that impact cell migration and wound healing. Although Tcf3 is induced at the wound edge and its overexpression can promote cell migration and wound repair, ablation of Tcf3 alone does not result in defective wound repair (data not shown). Since Tcf4 is also induced at the wound edge, can promote cell migration in vitro and can also induce Lcn2 ( Supplementary Figs 1,3 and Fig. 6c ), it is most likely that Tcf4 can compensate for the loss of Tcf3. Moreover, since Lcn2 is known to be upregulated by other factors (proinflammatory cytokines IL1β, IL17, and TNFα and other transcriptional factors such as NF-κβ, NFAT1 and C/EBPβ) [37] , [64] , it is not surprising to find that loss of Tcf3 is not sufficient to result in either a significant reduction in the level of Lcn2 or a consequent reduction in wound repair. Together, these results suggest a model that defines a molecular genetic axis in wound-repair in which Stat3 is required for the induction of Tcf3, which through its repressor function, leads to the secretion of Lcn2 to promote wound repair through a cell migration mechanism ( Fig. 10 ). While Stat3 and Lcn2 have been shown to play a role in cell migration, Tcf3’s role in cell migration was unknown. Our findings are the first to demonstrate a relationship between Stat3, Tcf3 and Lcn2 in wound repair. Our results also show a novel role for Tcf3 and Lcn2 in epidermal cell migration and skin wound healing and provide a potential target for development of new treatments for defective wound repair. 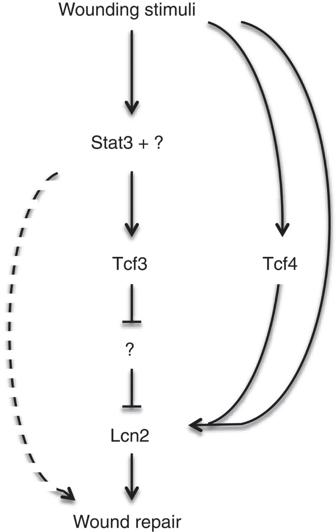Figure 10: Model depicting Stat3-Tcf3-Lcn2 axis in wound healing. This study shows that Tcf3 induction in response to wounding is dependent on Stat3 and that Lcn2 is Tcf3’s downstream effector that promotes cell migration and wound repair. While Tcf3 is sufficient for the induction of Lcn2, it is not absolutely required, most likely because Tcf4 can compensate for Tcf3, as it does in other skin-related phenotypes, or because additional factors can induce Lcn2. While Lcn2 is necessary and sufficient for proper wound repair, it does not fully explain how the loss of Stat3 impacts wound repair, because Tcf4 induction is not controlled by Stat3 and Lcn2 application on Stat3 cKO wounds does not fully rescue the repair defect. Figure 10: Model depicting Stat3-Tcf3-Lcn2 axis in wound healing. This study shows that Tcf3 induction in response to wounding is dependent on Stat3 and that Lcn2 is Tcf3’s downstream effector that promotes cell migration and wound repair. While Tcf3 is sufficient for the induction of Lcn2, it is not absolutely required, most likely because Tcf4 can compensate for Tcf3, as it does in other skin-related phenotypes, or because additional factors can induce Lcn2. While Lcn2 is necessary and sufficient for proper wound repair, it does not fully explain how the loss of Stat3 impacts wound repair, because Tcf4 induction is not controlled by Stat3 and Lcn2 application on Stat3 cKO wounds does not fully rescue the repair defect. Full size image Mice Tet-inducible Tcf3 mice were generated by crossing K14-rtTA with TRE-Tcf3 (ref. 22 ). Intercrosses between the Stat3 fl/fl line [30] and K14-Cre (Jackson Laboratory) were done to yield Stat3 cKO mice. Intercrosses between the Tcf3 fl/fl line [23] and K14-Cre yielded Tcf3 cKO mice. Lcn2 KO mice were obtained from Dr S. Akira [58] . Tet-inducible Stat3C transgenic mice were generated by crossing K14-rtTA with TRE-Stat3C . The XhoI and DrdI fragment of pTRE-Stat3C was microinjected into pronuclei of FVB/N embryos to generate the TRE-Stat3C transgenic line. All mice were maintained in the AALAC-accredited animal facility at Baylor College of Medicine and were used according to protocols that were approved by the Baylor College of Medicine institutional care and use committee. In vivo wound closure assay For wounding experiments, 8- to 10-week-old Stat3 cKO ( Stat3 fl/fl ;K14-Cre ) or control ( Stat3 fl/f ) female mice were anesthetized with intraperitoneal administration of ketamine/xylazine and full-thickness wounds were made on the mid dorsal skin with 4-mm disposable biopsy punches. Skins were harvested and embedded in OCT (Tissue-Tek) 3, 5 or 7 days post wounding. To evaluate the effect of Tcf3 expression on wounds repair, full thickness wounds of 1 cm 2 were created on the dorsal skins of Tcf3 inducible ( K14-rtTA;TRE-mycTcf3) or control ( K14-rtTA or TRE-mycTcf3 ) mice, which had been maintained on Dox (200 mg kg −1 ) containing chow (Bio-Serv) for 6 months starting at 8 weeks of age. Skins were harvested and embedded in OCT 6 or 10 days post wounding. To evaluate the effect of conditioned media (CM) from Tcf3- or Lcn2-overexpressing cells on wound closure, full-thickness wounds of 1 cm 2 were created on the dorsal skins of 8- to 10-week-old ICR mice. A quantity of 200 μl of CM was topically applied onto the wound sites and the surface areas of the wounds were measured. Each wound was covered with Tegaderm film and a self-adherent wrap (Coban) to prevent leakage, desiccation and infection. CM was generated by feeding 80–90% confluent keratinocytes in 15-cm tissue culture plates with 18 ml per plate serum-free MCDB153 medium and incubating for 48 h. The CM was concentrated 20-fold by using Amicon centrifugal filter units with a 10-kDa cut-off (Millipore) following the manufacturer’s instructions. The concentrated CM was mixed with carboxymethylcellulose solution (final concentration, 3% w/v) before being topically applied onto the wound bed. To evaluate the effect of recombinant Lcn2 on wound closure, 200 μl of Lcn2 (R&D Systems), dissolved at 1 μg ml −1 in PBS containing 3% carboxymethylcellulose was applied onto the wound bed and wound closure was evaluated as described above. To evaluate the depletion of Lcn2 on wound healing, 200 μl of 3 μg ml −1 anti-Lcn2 (R&D Systems) or goat IgG in PBS containing 3% carboxymethylcellulose were applied every other day for 11 days to 1 cm 2 wounds that were created on 4-month-old female athymic nude mice. To evaluate whether recombinant Lcn2 can rescue defective wounding healing in Stat3 cKO mice, 1 cm 2 wounds were created on dorsal skins of Stat3 cKO ( Stat3 fl/fl ;K14-Cre ) or littermate controls (Stat3 fl/fl ) that were waxed for 2 weeks prior to wounding. A quantity of 200 μl of 2 μg ml −1 EGF (Invitrogen) with or without recombinant 2 μg ml −1 of Lcn2 in PBS +3% carboxymethylcellulose were applied to the wound beds every other for 11 days. Wound closure was evaluated as described above. Ex vivo skin explant outgrowth assay Ex vivo explant culture of 2- to 4-day-old mouse skin was carried out as previously reported [65] , [66] . Briefly, circular skin biopsies were obtained from dorsal skin of 2-day-old female and male pups of the same litters using 4-mm biopsy punches (Sklar) and were plated with 0.3-ml medium on 24-well plates (BD Biosciences). After overnight incubation at 37 °C, 7.5% CO2, explants were submerged in media with or without Dox (1 μg ml −1 ) and grown for another 8 days before fixing (4% paraformaldehyde (PFA) for 10 min; 100% methanol for 10 min at −20 °C). Medium was changed every 2–3 days. In cases of mitomycin C treatment, skin explants were treated with 8 μg ml −1 mitomycin C (Roche) 48 h post Dox treatment. After mitomycin C treatment, cultures were washed three times with PBS and refed with fresh media. Keratinocytes in the cellular outgrowth of explants were identified by immunostaining for Keratin 17 and by morphological appearance. Images of the cellular outgrowth from each explant were taken, and the proximal distance extending between the explant biopsy and the distal edge of the cellular migration was measured using NIH ImageJ software ( http://rsb.info.nih.gov/ij/ ). Measuring the surface area covered by the keratin 17-positive outgrowth yielded similar findings. Plasmid constructs Gateway entry vectors for the Lef/Tcf genes of interest were generated as follows: The myc-tagged Tcf3 wild-type and mutant alleles [20] were PCR-amplified from their respective vectors with the addition of Eco RI and Xho I sites with primers myctag_EcoRI_fw and Tcf3 Δ C_XhoI_rv2 (for Tcf3ΔC ) or Tcf3_XhoI_rv (for the others). The PCR was conducted using Phusion DNA polymerase (New England Biolabs, Ipswich, MA). The resulting PCR products were then subcloned into pENTR 1 A (Life Technologies, Carlsbad, CA). Myc-tagged Tcf4 was subcloned from K14-mycmTcf4 (ref. 23 ) into pENTR 1 A by Bam HI/ Not I digest. Myc-tagged Lef1 was subcloned from K14-mycmLef1 (ref. 67 ) into pENTR 1A by Eco RI/ Xba I digest. To clone myc-tagged Tcf1 , total RNA was TRIzol-purified from adult C57BL/6 mouse splenocytes and reverse-transcribed into cDNA using SuperScript III reverse transcriptase (Life Technologies, Carlsbad, CA) with oligo(dT) 20 primers. The full-length Tcf1 ORF (from NM_009331) was PCR-amplified, with the addition of Eco RI and Not I sites and a myc tag, using the primers mTcf1_myc_Eco_fw and mTcf1_Not_rv. The PCR was conducted using Herculase II polymerase (Agilent Technologies, Santa Clara, CA). The resulting PCR product was digested and subcloned directly into Eco RI/ Not I-digested pENTR 1A. A negative-control entry vector was generated by digesting pENTR 1A with Eco RI and recircularizing it. To generate Tet-inducible lentivirus constructs, the Gateway entry vectors were recombined into pINDUCER21 (ref. 27 ) using LR Clonase II (Life Technologies, Carlsbad, CA) according to the manufacturer’s instructions. Tcf3pro- luc constructs were generated by PCR from mouse embryonic stem cell genomic DNA. 4884, bp of the proximal Tcf3 promoter was amplified with primers to introduce an Mlu I site at the 5′ end and an Xho I site at the 3′ end. The fragment was then subcloned into the pGL3-basic vector (Promega). Site-directed point mutation of Tcf3 promoter for Stat3 binding sites was made as reported [68] . Two PCR reactions were performed in parallel using the methylated parental Tcf3pro- luc plasmid and either forward or reverse primer carrying the mutation. The products from the two PCR reactions were combined. After being heated at 95 °C, the PCR product mixture was cooled down to allow random annealing of the PCR products with parental strands. The mixture was treated with DpnI to digest methylated, non-mutated parental strands and then transformed to competent cells. pTRE-Stat3C was engineered as follows: the β -globin intron was subcloned from the K14 cassette vector (Elaine Fuchs lab) into the SacII site of pTRE2 (Clontech) to form the vector pTRE2I . The Stat3C-Flag ORF from the pBabe-Stat3C expression vector (a gift from Dr. Jacqueline Bromberg of MSKCC) was digested with BamHI , then ligated into the BamHI site of pTRE2I . All plasmids were verified by restriction digest and sequencing before use. All cloning primers are listed in Supplementary Table 1 . Lentivirus production 293T cells were cultured in IMDM containing 10% fetal bovine serum (FBS), 2 mM Supplementary L -glutamine, and pen/strep. To produce lentivirus particles, cells were plated at 4 × 10 6 cells per 10 cm plate. The following morning, they were transfected with 7 μg pINDUCER vector and 750 ng each of pHDM-Hgpm2, pRc/CMV-RaII, pHDM-tat1b and pHDM-VSV-G with 30 μl of TransIT-293 transfection reagent (Mirus Bio) per 10 cm plate. Twenty-four hours after transfection, media was changed and volume reduced to 6 mL per 10 cm plate. Virus-containing supernatants were collected at 48 and 72 h post transfection, pooled and concentrated by ultracentrifugation at 85,000 g for 2 h. Virus particles were resuspended in a small amount of keratinocyte growth media, separated into aliquots and stored at −80 °C until use. Virus preps were titered by infection of 293T cells with 10-fold serial dilutions of lentivirus followed by flow cytometric analysis for GFP positivity. Titres (in transduction units per microliter) were calculated using the formula ((fraction GFP positive)(number of cells at time of infection))/((dilution factor)(volume of viral inoculum)). Keratinocyte culturing and lentiviral infection Primary keratinocytes were isolated as described [22] . Dorsal skins were dissected from newborn pups and put on 1 U ml −1 dispase I solution (with the epidermis side upward) at 4 °C for overnight. After 16–20 h, the epidermis was peeled off and immediately placed on 0.05% trypsin for 5 min, followed by vigorously pipetting to separate basal layer cells. After being filtered through a 40 μm cell strainer, primary keratinocytes were cultured on J2 fibroblasts treated with mitomycin C (Roche) for three passages before being cultured without feeder cells. For lentiviral infections, keratinocytes were plated at 1 × 10 5 cells per well in 6-well tissue culture plates. The following day, one or two representative wells were trypsinized and counted. Lentivirus preps were thawed and diluted in keratinocyte growth media containing 8 μg ml −1 Polybrene (Sigma-Aldrich, St Louis, MO), to a final multiplicity of five transduction units per cell. Growth media was aspirated from the plated keratinocytes and replaced with diluted lentivirus (1 mL per well). The plates were incubated at 37 °C for 15 min and then centrifuged at 1,100 × g, 32 °C, for 30 min. After centrifuging, the cells were washed with 3 ml per well PBS, refed with keratinocyte growth media, and returned to 37 °C for growth. GFP expression was detectable 72 h following infection. For the cell proliferation assay, 2 × 10 4 cells were plated onto each well of a 24 well plate. Cells were trypsinized and counted in triplicates using a Beckman Z2 Coulter counter every 24 h. Flow cytometry After lentiviral transduction, cells were grown to confluence, and then sorted by flow cytometry. Cells were trypsinized, then resuspended in ice-cold sorting buffer (4% calcium-free chelated FBS in PBS, ~200–300 μm per 10 cm plate), and strained into 30 μm strainer-cap FACS tubes and kept on ice. Cells were isolated on a FACSAria II or IIu cell sorter (BD Biosciences), using the 100 μm nozzle at a sheath pressure of 20 psi. GFP positives (typically 60–80% of cells) were collected in chilled 15 ml catch tubes containing 6 ml of keratinocyte growth media. After collection, cells were pelleted, resuspended, counted and replated for growth in keratinocyte growth media. In vitro wounding assay The in vitro wounding assay was performed as described [2] , [26] with some modifications. Keratinocytes were cultured in 6-well plates until reaching confluence. They then were starved in serum-free basal medium with or without Dox for 22 h, followed by treatment with 10 μg ml −1 mitomycin C for 2 h. After creating a straight scratch with a pipette tip, the cells were washed three times with PBS to remove mitomycin C and cell debris. For testing functions of various genes in cell migration, the cells were refed with serum-containing medium with or without Dox, and cell migration was stopped 14–16 h later by fixing with 3.8% PFA. Alternatively, in the rescue experiments, following starvation, mitomycin C treatment and scratching, the cells were incubated in basal medium complemented with 10 ng ml −1 mouse recombinant EGF (Invitrogen, United States) with or without Dox. Immediately after a scratch was created, markings were made adjacent to the scratch as a reference for camera positioning. Photographs were taken at the initial and final time points using a phase-contrast microscope (Axiovert 40; Zeiss, Germany). By comparing the images from initial to final time points, the area filled by migrating cells was quantified with ImageJ analysis software ( http://rsb.info.nih.gov/ij/ ). For each sample, over 30 non-overlapping fields were measured at each time point; and each experiment was repeated at least twice. Values represent the mean±s.d. of migrated area beyond the edges of the scratch. Luciferase reporter assay pBabe-Stat3 and pBabe-Stat3C expression vectors were gifts from Dr Jacqueline Bromberg (Memorial Sloan-Kettering Cancer Institute). For the reporter assay, keratinocytes were plated at density of 2 × 10 4 cells per well in a 24-well plate 1 day before transfection. The Tcf3 pro-luc, Tcf4 pro-luc and the Stat3 expression vector, along with the control vector pRL-TK were transfected using FuGENE 6 (Roche) according to the manufacturer’s instructions. Luciferase reporter activity was measured using the Dual-Luciferase Reporter system 48 h after transfection (Promega) with Firefly luciferase values normalized to Renilla luciferase values. Real-time PCR Total RNA was purified with the ZR RNA Miniprep kit (Zymo Research, Irvine, CA) and 1 μg of each RNA sample was reverse transcribed with the Superscript III First-Strand Synthesis System (Life Technologies, Carlsbad, CA) using Oligo(dT) primers. PCR amplifications of genes of interest were performed using primers located in different exons or spanning intron–exon junctions to obtain amplicons less than 150 bp in length. Real-time PCR was performed with LightCycler DNA Master SYBR Green I reagents on a LightCycler 480 real-time PCR system (Roche, United States). Differences between samples and controls were calculated based on the 2 −ΔΔCP method, using the Mrpl19 gene as an internal control. Primer sequences are listed in Supplementary Table 1 . Immunohistochemistry and immunofluorescence For immunohistochemical detection, 5 μm paraffin sections were used; and endogenous biotin and peroxidase activity were blocked. The colour was developed with DAB chromogen (ImmPACT DAB; Vector Laboratories, United States) and the sections were counterstained with hematoxylin. Immunofluorescence analysis was performed as described [22] . A total of 6–8 μm frozen back skin sections were fixed in 4% PFA. For blocking, the MOM kit (Vector Laboratories, Burlingame, CA) was used for mouse monoclonal antibodies, and the following blocking buffer for all other antibodies: 10% normal donkey serum, 2% BSA, 2% fish skin gelatin, 2% Triton X-100 in PBS. Primary antibodies were used at the following concentration: guinea pig anti-Tcf3 (1:200, lab-generated), rabbit anti-Tcf4 (1:200; Cell Signalling), rabbit anti-Tcf1 (1:50; Cell Signalling), rabbit anti-Lef1 (1:150; Cell Signaling), mouse anti-myc tag (1:500; Zymed), mouse anti-β-catenin (Sigma), mouse anti-Stat3 (1:300; Cell Signaling), pY705-Stat3 (1:100; Cell Signaling), rat anti-cd104 (1:200; BD Biosciences) goat anti-Lcn2 (1:150;R&D Systems). Antigens were visualized with FITC- or RRX-conjugated secondary Abs (Jackson Labs). All images were acquired with Zeiss Axioskop microscope. Protein extraction Cultured cells were lysed with RIPA buffer supplied with protease inhibitor cocktail (Roche). Biopsies of wounded or unwounded skin were homogenized with beads in 1-ml TRI Reagent and total proteins were extracted according to the reagent’s protocol (Life Technology). The protein precipitates were resolved in the solvent consisting of 4 M urea, 0.5% SDS and 5 mM DTT, with concentrations over 2 mg ml −1 . Protein concentrations were determined with the Bradford Protein Assay kit (Pierce). Immunoblot and in situ hybridization To analyse tet-inducible gene expression, 40 μg protein from the total cell lysate of lentivirus-transduced keratinocytes was resolved by SDS–PAGE. The separated proteins were then immunoblotted, probed with primary myc tag antibody (1:3,000, Abcam), and detected by chemiluminescence (SuperSignal West Pico, Thermo Scientific). The in situ hybridization was carried out as described previously [69] . Five days post wounding back skins of 8- to 10-week-old wild-type and Stat3 cKO mice were frozen side by side in Tissue-Tek OCT reagent, and cryo-sections (16 μm) were prepared. The sections were fixed in 4% formaldehyde in PBS and acetylated, followed by prehybridization. Probes used were DIG-labelled (Roche) sense and anti-sense transcripts of mouse cDNAs of Tcf3 (NM_001079822, nucleotides 1-1030). After hybridization, sections were treated with RNase A and extensively washed. The DIG-label was detected by an anti-DIG Fab (Roche) coupled to alkaline phosphatase using NBT/BCIP (Roche) according to the manufacturer’s instructions. Sections were then counterstained with nuclear fast red (Vector Laboratories). ELISA Lcn2 levels were determined with the Lcn2 quantikine kit (R&D Systems). Conditioned media were diluted × 20 with the RD5-24 diluent before being loaded. For quantification of Lcn2 in the skin extracts, the protein samples were diluted to 0.2–0.5 pg μl −1 . The standard protein dilutions were made in the solution containing the same concentration of total proteins extracted from Lcn2 KO skin to improve the recovery rate to over 80%. The linearity-of-dilution reached ~100%. Chromatin immunoprecipitation ChIP was performed according to the manufacturer’s protocol (Upstate Biotechnology) with modifications. Hair follicle cells were isolated from P4 mouse pups as described [69] . The dorsal skins were incubated with 1 U ml −1 dispase for 50 min at 37 °C to separate the dermis from the epidermis. The dermis was cut into small pieces and then incubated with collagenase for ~40 min at 37 °C. The hair follicles were further dissociated from the surrounding dermis with a mild swirling shearing stress in fluid, and enriched by centrifugation at 20 g . After the hair follicles were disintegrated by trypsinization, the cells were dispersed, filtrated and directly fixed with 1.42% formaldehyde in 4% FBS–PBS solution at room temperature for 15 min. Cross-linked DNA was sonicated to form fragments ranging from 200–500 bp in length. After preclearing, ChIP lysates were immunoprecipitated with rabbit anti-Stat3 (Cell Signaling), and rabbit IgG (Jackson Laboratory). Pulled-down DNA fragments were recovered with the Chelex-100-mediated purification method [70] . Conserved Stat3 sites identified by rVista analysis of 5′ upstream sequences were defined by the ECR Browser and Ensembl software. Stat3 sites were chosen for ChIP analysis based on the conservation and alignment between mouse, rat and human. qPCR was done with the LightCycler 480 system (Roche, United States) using the PerfeCTa SYBR Green FastMix kit (Quanta Biosci) and primers to produce amplicons less than 150 bp. Primer sequences are listed in Supplementary Table 1 . The ChIP on skin tissue was performed according to the manufacturer’s protocol (Cell Signaling Technology) with modifications. The dorsal skins of 8-week-old ICR mice were wounded using 4-mm biopsy. Five days later, the wound edge (~1 mm) and adjacent skin (as the unwounded control) were dissected and flash frozen in liquid nitrogen. About 200 mg of the skin tissue was cryogenically ground in liquid nitrogen in a mortar. Then the tissue powder was transferred to 50-ml tubes for fixation in fresh 1.5% formaldehyde in 1 × PBS for 30 min at room temperature. After being quenched with 0.125 M glycine, then rinsed twice with PBS, the tissue was resuspended in PBS and dounce-homogenized. The cell suspension was aliquoted into three 1.5-ml Eppendorf tubes and stored at −80 °C prior to use. Cells were lysed in swelling buffer (5 mM PIPES, pH8, 85 mM KCl, 0.5% NP40), and sheared in sonication buffer (50 mM Tris–HCl, pH 8.1, 1% SDS, 10 mM EDTA) for 9 × 30 s pulses (90 s pause between pulses) using a Misonix Sonicator 3000. After sonication, the lysates were cleared by centrifugation at 16,000 g for 10 min. One-twentieth volume of the supernatant was used to analyse chromatin shearing and concentration. Approximately 7 μg of the cross-linked chromatin was diluted 10-fold into ChIP dilution buffer (20 mM Tris–HCl, pH 8.1, 0.01% SDS, 1% Triton X-100, 2 mM EDTA, 150 mM NaCl), and incubated with mouse anti-Stat3 monoclonal antibody (Cell Signaling) or mouse IgG (Jackson Laboratory) overnight. Then the sample was mixed with 30 μl of Dynabeads Protein G that had been washed with block solution (1 × PBS, 0.5% BSA) and rotated for 2 h before magnetic separation. Beads were washed 2 × with 20 mM Tris–HCl (pH 8), 0.1% SDS, 1% Triton X-100, 2 mM EDTA, 150 mM NaCl, 1 × with 10 mM Tris–HCl (pH 8), 250 mM LiCl, 0.5% NP40, 0.5% deoxycholate, 1 mM EDTA and 1 × with TE containing 50 mM NaCl. Bound complexes were eluted with the Chelex-100-medited purification method. Statistical analysis Statistical analyses were performed using Microsoft Excel. The Student’s t -test function with a two-tailed distribution was used to calculate P -values. Differences were regarded as statistically significant and as statistically highly significant if P -values were <0.05, and P <0.001, respectively. How to cite this article : Miao, Q. et al . Tcf3 promotes cell migration and wound repair through regulation of lipocalin 2. Nat. Commun. 5:4088 doi: 10.1038/ncomms5088 (2014).